The rediscovered Hula painted frog is a living fossil Amphibian declines are seen as an indicator of the onset of a sixth mass extinction of life on earth. Because of a combination of factors such as habitat destruction, emerging pathogens and pollutants, over 156 amphibian species have not been seen for several decades, and 34 of these were listed as extinct by 2004. Here we report the rediscovery of the Hula painted frog, the first amphibian to have been declared extinct. We provide evidence that not only has this species survived undetected in its type locality for almost 60 years but also that it is a surviving member of an otherwise extinct genus of alytid frogs, Latonia , known only as fossils from Oligocene to Pleistocene in Europe. The survival of this living fossil is a striking example of resilience to severe habitat degradation during the past century by an amphibian. The Hula painted frog was described as Discoglossus nigriventer (Mendelssohn and Steinitz [1] ) in the early 1940s following the discovery of two adults and two tadpoles in a freshwater habitat on the eastern part of the Hula Valley (Israel, 33°6′12"N, 35°36′33"E). An additional single adult collected in 1955 during the drainage of the Hula Valley wetlands was the last confirmed sighting of this species [2] despite numerous later surveys. In 1996, this frog was the first amphibian species to be declared by the IUCN as extinct [3] , [4] , [5] . Considering concerns on global amphibian decline [6] , this species was selected as one of the ‘top 10’ species during the ‘Search for Lost Frogs’ initiative by Conservation International ( www.conservation.org ), and became a poignant symbol of extinction for Israel. Within its family, the Alytidae, the Hula painted frog is unique in its east Mediterranean distribution. To date, all records indicate that the species is endemic to the Hula Valley in northern Israel. Alleged records from a marsh south of the Lebanese Beqaa Valley (Lebanon, 34°00′54"N, 36°10′36"E) remain unconfirmed [7] . In October 2011, a routine patrol in the Hula Nature Reserve discovered an adult male unambiguously identified as a Hula painted frog ( Fig. 1 ) at midday, in a terrestrial habitat, ca. 10 m from a 0.05-km 2 pond. Since then, we have recorded 10 more specimens (five males, one female and four juveniles) all within a restricted area of about 1.25 ha. Seven of these were located in terrestrial habitat, beneath a ca. 20 cm layer of wet detritus, within a dense growth of reeds ( Phragmites australis ) and blackberry ( Rubus sanguineus ). Three other individuals were collected while being taken by kingfishers ( Halcyon smyrnensis ). 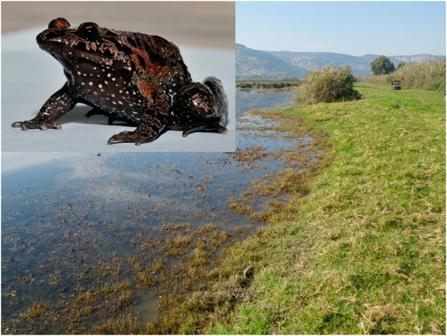Figure 1: Lateral and ventral view of a femaleL. nigriventer. In the background, the typical habitat in the Hula reserve where extant individuals have been found (photographs by Frank Glaw). Figure 1: Lateral and ventral view of a female L. nigriventer . In the background, the typical habitat in the Hula reserve where extant individuals have been found (photographs by Frank Glaw). Full size image In the 1960s, a probable Hula painted frog fossil bone was reported from an Early Pleistocene site, ‘Ubeidiya’ in the Jordan Valley, Israel [8] . Since then, more Alytidae fossils were recovered from three Pleistocene archaeological sites in the Hula Valley [9] : the Early-Middle Pleistocene site of Gesher Benot Ya'aqov [10] , and two Late Pleistocene sites, Nahal Mahanayeem Outlet [11] and Ain Mallaha/Eynan [12] ( Supplementary Note 1 ). Here we report on the taxonomic status of the recently rediscovered Hula painted frog. Our molecular analyses show that the Hula painted frog is a sister group to a clade containing all other species of Discoglossus . Based on osteological characters, all the fossils from the Hula Valley are similar to the contemporary Hula painted frog. Furthermore, the osteology of the Hula painted frog shares more apomorphic morphological characters with Latonia, a widespread European clade from the Oligocene–Pleistocene eras, than with any Discoglossus species. In other words, the Hula painted frog is a living fossil, and therefore calls for special attention to its survival. Molecular analysis We sampled tissue from six of the specimens collected during 2011. We sequenced a total of 2,503 bp DNA from three nuclear and three mitochondrial genes, yielding a mean (±s.d.) intraspecific nucleotide divergence per gene of 0.005±0.003, which implies low genetic divergence among individuals. Maximum likelihood and Bayesian inference phylogenetic trees ( Fig. 2a , Supplementary Fig. S1 ) confirm the Hula painted frog as belonging to the family Alytidae, an ancient Old World anuran clade that together with its sister group, the Bombinatoridae, originated deep in the Jurassic [13] and currently contains a total of only 12 species [14] . All our analyses strongly support the Hula painted frog being the sister group to a clade containing all other species of Discoglossus whose relationships are recovered congruent with other studies [11] . Molecular time-trees obtained by relaxed-clock approaches date the origin of this frog deep into the tertiary. Analyses were calibrated primarily with time constraints related to the vicariance of Iberian and North-African alytids at 5 mya, after the Messinian salinity crisis [15] , given that our phylogenetic analyses recovered sister-group relationships among the taxon pairs Discoglossus scovazzi (Morocco) and Discoglossus galganoi/jeanneae (Iberia), and Alytes maurus (Morocco) and Alytes dickhilleni (Iberia). Additional time constraints used after cross-validation were secondary calibrations of 152 mya for the split between Alytidae and Bombinatoridae, 10 mya for the split between Bombina orientalis and B. bombina , and a root prior of 240 mya. According to our preferred estimate (allowing substitution rates to vary independently over clades, and based on nuclear DNA only) and the combined 95% credibility intervals from various analysis methods, the split of the Hula painted frog from the western Discoglossus species took place at about 32 mya (19-70 mya), probably during the Late Eocene or Early Oligocene ( Fig. 2b ). Cladogenesis among the western Discoglossus species occurred from about 16 mya onwards, in agreement with previous estimates [14] . Additional analyses including partial sequences of Barbourula confirm placement of this Asian genus sister to Bombina in the Bombinatoridae [16] and distant to the Hula painted frog ( Supplementary Figs S2 and S3 , Supplementary Table S1 ). 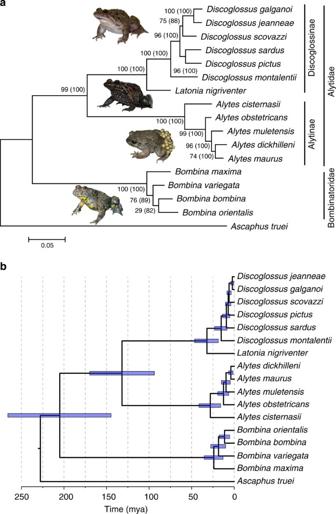Figure 2: Molecular phylogeny of recent Alytidae and Bombinatoridae. (a) Maximum likelihood tree based on 2,503 bp DNA sequences from six different genes, showing the position ofL. nigriventersister toDiscoglossus.Ascaphus truei(Ascaphidae) was set as outgroup. Values on nodes are the bootstrap support for the maximum likelihood phylogeny, and the credibility values for the Bayesian phylogeny in percent (in parentheses). (b) Time tree for the Alytidae and Bombinatoridae. Confidence intervals for the nodes are indicated in purple. Figure 2: Molecular phylogeny of recent Alytidae and Bombinatoridae. ( a ) Maximum likelihood tree based on 2,503 bp DNA sequences from six different genes, showing the position of L. nigriventer sister to Discoglossus . Ascaphus truei (Ascaphidae) was set as outgroup. Values on nodes are the bootstrap support for the maximum likelihood phylogeny, and the credibility values for the Bayesian phylogeny in percent (in parentheses). ( b ) Time tree for the Alytidae and Bombinatoridae. Confidence intervals for the nodes are indicated in purple. Full size image Morphological analysis We examined Hula painted frog osteology using microtomography scans of four individuals (one collected in 1955 and three in 2011). The Hula specimens (including the Pleistocene fossils) display general discoglossine features following previous morphological analyses [17] , [18] , [19] . However, they share certain distinct morphological characters exclusively with the fossil genus Latonia and not with western Discoglossus . All Hula painted frogs (recent and fossil) have a double coronoid process on the angular ( s. l. ), an apomorphic character ( Fig. 3 ) that differentiates Latonia species from other anuran amphibians, western Discoglossus included [17] , [18] . Additional characters common to Latonia and the Hula painted frog, but absent in Discoglossus , are as follows: (1) Pterygoid with a well-developed ventral flange, (2) Maxilla with a long, horizontal and linear dorsal margin of the zygomatico-maxillary process, (3) Well-developed pterygoid process of the maxilla, (4) Posterior depression on the inner surface of the maxilla and (5) Angular ( s. l. ) with flat, enlarged and delimited upper margin of its postero-lateral wall. 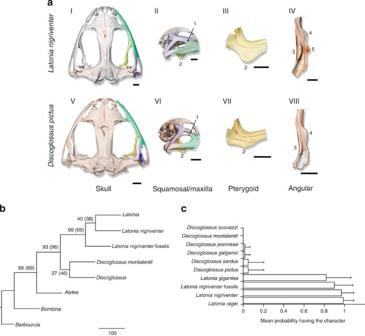Figure 3: Osteological relationships of recent and fossil Alytidae. (a) Diagnostic osteological characters distinguishingL. nigriventerandDiscoglossus pictus. For both species, we show the skull in dorsal view (I, V), lateral views of squamosal and maxilla (II, VI) and the pterygoid (III, VII), and a dorsal view of the angular (IV, VIII). The maxilla is indicated in green, pterygoid in yellow and the squamosal in blue. The numbered lines denote the squamosal—maxilla articulation (1), ventral flange of the pterygoid (2), the upper margin of the postero-lateral wall of the angular (3), the anterior coronoid process (4) and the posterior coronoid process (5). (b) Phylogeny of Alytidae based on 22 osteological characters (Bombinatoridae were used as outgroups). Values on nodes are the bootstrap support for the most parsimonious phylogeny, and the credibility values for the Bayesian phylogeny (in parentheses), both in percent. (c) Mean (±s.d.) probability of character presence. Probabilities were calculated using a logistic regression (Likelihood ratio test: speciesχ92=157.4,P<0.0001, characterχ92=8.2,P=0.510 and species* characterχ752=38.8,P<=0.999). Bold letters denote fossil species. Scale bars, 2 mm. Figure 3: Osteological relationships of recent and fossil Alytidae. ( a ) Diagnostic osteological characters distinguishing L. nigriventer and Discoglossus pictus . For both species, we show the skull in dorsal view (I, V), lateral views of squamosal and maxilla (II, VI) and the pterygoid (III, VII), and a dorsal view of the angular (IV, VIII). The maxilla is indicated in green, pterygoid in yellow and the squamosal in blue. The numbered lines denote the squamosal—maxilla articulation (1), ventral flange of the pterygoid (2), the upper margin of the postero-lateral wall of the angular (3), the anterior coronoid process (4) and the posterior coronoid process (5). ( b ) Phylogeny of Alytidae based on 22 osteological characters (Bombinatoridae were used as outgroups). Values on nodes are the bootstrap support for the most parsimonious phylogeny, and the credibility values for the Bayesian phylogeny (in parentheses), both in percent. ( c ) Mean (±s.d.) probability of character presence. Probabilities were calculated using a logistic regression (Likelihood ratio test: species χ 9 2 =157.4, P <0.0001, character χ 9 2 =8.2, P =0.510 and species* character χ 75 2 =38.8, P <=0.999). Bold letters denote fossil species. Scale bars, 2 mm. Full size image Phylogenetic analyses on 22 morphological characters from contemporary and fossil Alytidae using a variety of approaches (trees based on morphology alone, and combining morphological and molecular characters) consistently recover a clade containing contemporary and fossil Hula painted frogs, and Latonia fossils, with highest support values for this clade after exclusion of those fossil taxa for which many morphological data are missing ( Fig. 3b , Supplementary Figs S2 and S3 , Supplementary Table S2 , Supplementary Note 2 ). None of the remaining fossil Alytidae or Bombinatoridae are placed within or sister to this clade in any analysis, in agreement with previous reconstructions [20] . Logistic regression analysis on bones of recent and fossil Hula painted frogs, Latonia fossils, and recent Discoglossus species confirms the clustering of the Hula painted frog with Latonia, and not with any of the Discoglossus species ( Fig. 3c ; Supplementary Table S3 ). The Hula painted frog also differs externally from Discoglossus . The black abdomen, dotted with white spots each corresponding to a wart, is typical only to this species, whereas a white abdomen characterizes all other Discoglossus species. A deep transversal fold, discernible on the neck of Latonia nigriventer , is not typical to any Discoglossus species, nor found in other Alytidae. Although not reaching the giant sizes of fossil Latonia [17] , [18] (snout-to-vent length (SVL) up to 200 mm), this species is the largest of all extant Alytidae with up to 84 mm in SVL and 53 g in weight (>100 mm SVL in Hula Valley fossils), compared with exceptional maximum sizes of 75–80 mm SVL in the other painted frogs. Differences in external morphology and osteology thus confirm Latonia and Discoglossus as two distinct sister genera of deep molecular divergence and reciprocal monophyly. Overall, the above morphological and molecular results strongly support the Hula painted frog as not being a species of Discoglossus as previously considered, but as the only living representative of the osteologically well-diagnosable fossil genus Latonia . We therefore propose its transfer to this genus as L. nigriventer (Mendelssohn and Steinitz [1] ) comb. nov. In other words, the Hula painted frog is a living fossil. This conclusion may also be supported by the spatial distribution of these genera. Fossils and extant species of Discoglossus are found mainly in the western Mediterranean region (western Europe and western North Africa), whereas Latonia fossils occur throughout Europe, including the Anatolian and Balkan peninsulas at the eastern Mediterranean ( Fig. 4 ). During the Pleistocene, Latonia fossils abruptly disappeared from European sediments (last recorded from the Early Pleistocene, Calabrian stage, at Pietrafitta in Italy [21] ), an extinction presumably caused by continental glaciations [22] . Latonia was probably present in the Middle East before the onset of the Pleistocene. The fossil record shows that during the Miocene, Latonia was widespread throughout Europe, reaching eastwards to Turkey [22] ( Fig. 4 ). We hypothesize that during this period Latonia reached and colonized the Middle East, including the Hula Valley in Israel. 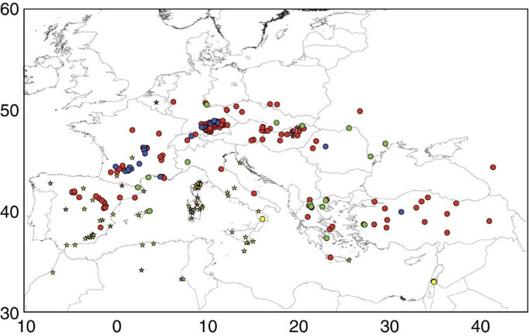Figure 4: Distribution of Discoglossinae fossils in Europe. Shapes denote genera (star=Discoglossus, circle=Latonia), and colours denote geological periods (red=Miocene, blue=Oligocene, green=Pliocene, yellow=Pleistocene and grey=Holocene). A few specimens were omitted from the map or their position is questionable (Supplementary Note 3). The distribution map was created based on three different databases (http://rocek.gli.cas.cz/Tertianura.pdf)41,42. Figure 4: Distribution of Discoglossinae fossils in Europe. Shapes denote genera (star= Discoglossus , circle= Latonia ), and colours denote geological periods (red=Miocene, blue=Oligocene, green=Pliocene, yellow=Pleistocene and grey=Holocene). A few specimens were omitted from the map or their position is questionable ( Supplementary Note 3 ). The distribution map was created based on three different databases ( http://rocek.gli.cas.cz/Tertianura.pdf ) [41] , [42] . Full size image Our findings also have important implications for conservation of this species. To date, the Hula Nature Reserve (3.5 km 2 ) is the only site where extant L. nigriventer have been observed, moreover, restricted to a single pond. Much of the original Hula swamp (30 km 2 ) and lake (14 km 2 ) have been drained, and the localities on the east of the valley, where this species was collected during the 1940–1950s, have undergone severe habitat degradation because of agriculture, eliminating swamp habitat. This frog survived in a remarkably small range and persisted over the last 60 years in an intensively disturbed habitat, undetected despite repeated surveys. The survival of this living fossil is a striking example of resilience to severe habitat degradation during the past century by an amphibian, and may imply on the future survival of this species despite the threat resulting from restricted distribution [23] . Maintaining water and habitat quality at the Hula Nature Reserve, and further research into the natural history of this species, are essential to ensure its survival. Plans to reflood parts of the Hula Valley and restore the original swamp habitat are in place, which may allow expansion in population size and a secure future for the Hula painted frog. Molecular methods Hula painted frogs were collected in the Hula Valley during daytime by probing the banks of ponds and sifting through dead vegetation. Captured animals were measured, sampled for DNA and released. Dead individuals were preserved in ethanol for further analyses (Tel Aviv University collection; Am2572-4). DNA was sampled from toe clips of six L. nigriventer , and tissue samples from a single representative of each of the following taxa: D. galganoi, D. jeanneae (here treated as species but often seen as subspecies of D. galganoi [14] ) , D. montalentii, D. sardus, D. scovazzi, A. cisternasii, A. dickhilleni, A. maurus, A. muletensis, B. bombina, B. maxima and B. orientalis . DNA was extracted using proteinase K followed by standard phenol/chloroform protocol. We used published primers for three mitochondrial genes (mitochondrial DNA (mtDNA)): 12S rRNA [24] , [25] , 16S rRNA [24] and cytochrome - b (ref. 26 ), and three nuclear genes (nuclear DNA (nDNA)): histone H3 (ref. 27 ), rhodopsin exon 1 (ref. 27 ) and recombination activating protein 1 [28] (details in Supplementary Table 4 ). PCR products were sequenced with an ABI 3100 automatic sequencer (Applied Biosystems). Sequence data for all other species were taken from published sources [29] . Overall, we compiled a total of 2,503 bp for 17 species ( Fig. 2 ), and 1140, bp of mtDNA for 21 species ( Supplementary Fig. S1 , Supplementary Note 4 ). We used maximum likelihood and Bayesian frameworks to reconstruct the phylogenetic position of L. nigriventer after determining from 28 possible substitution models the one best fitting our data (FindModel; http://darwin.uvigo.es/software/modeltest.html ) according to the Akaike Information Criterion (AIC). For the nDNA and mtDNA data sets, the best substitution model was General Time Reversible (GTR) plus Gamma (ΔAIC=25.8 between best and second best models). Maximum likelihood trees were inferred in MEGA 5.05 [30] , and 1,000 bootstrap replicates were calculated to assess the support of nodes. For the Bayesian phylogeny, we used MrBayes 3.1 (ref. 31 ). For all Bayesian analyses, we ran 10 [6] Markov chain Monte Carlo ( MCMC ) generations and sampled at a frequency of 100 (10,000 samples and 25% burn-in). We ensured that the s.d. of split frequencies was <0.01 and that potential scale reduction factor was about 1. Alternative analyses partitioning the combined molecular data set by either gene or codon resulted in topologies identical to the unpartitioned analysis and high support for all nodes. Specifically, partitioned Bayesian analyses were performed under two different partition schemes: (1) each gene as a separate partition except for 12S and 16S, which were defined as a single partition and (2) a set of seven partitions defining first, second and third codon positions of the three nuclear genes as three partitions (each merged for the three genes), the three codon positions of the mitochondrial cytochrome- b gene as one partition each, and the merged 12S and 16S sequences as one partition. Substitution models were separately determined for each partition. MrBayes analyses under these settings resulted in topologies identical to those of the unpartitioned analysis and had high support values for all nodes. Divergence time estimates Reconstruction of molecular time-trees was based on two different relaxed-clock approaches, either of which allows substitution rates to vary independently over clades (ICR; BEAST, with 50 (ref. 6 ) generations and a conservative burn-in of 10 [6] generations after examination of convergence of likelihood values and mixing of chains [32] ), or in an autocorrelated fashion (ACR: Multidivtime [33] ). All analyses were carried out separately for the concatenated mtDNA data set and the concatenated nDNA data set, and composite 95% credibility intervals were compiled from the two nDNA analyses [34] . We used substitution models as in the phylogenetic analyses, except for the nDNA-based BEAST analysis. In this latter analysis, we deviated from the complex GTR+I+G model suggested by AIC. Instead, we applied a simple Jukes–Cantor model to obtain a more realistic time estimate for some of the shallow splits, where only very few nDNA substitutions separated the terminals, and to achieve a better convergence of the posterior values. However, additional runs with GTR+I+G led to similar age estimates for the focal node, that is, the Latonia–Discoglossus split. Preferred analyses ran with all time constraints activated (as reported in results above), but additional runs were carried out to cross-validate these. The time constraints used for estimating divergence times of Discoglossus frogs were, on one hand, secondary constraints from a previous study [35] (with upper and lower bounds from previous 95% credibility intervals), and biogeographic constraints from sister group taxa occurring on opposite sites of the strait of Gibraltar. Time constraints (calibrations) in the following are named C0–C4: C0: We set the root prior in our analysis (split of Ascaphus from other frogs) at 240 mya [35] . C1: We used the constraint of 152 mya (129–179 mya) [35] for the split between Bombinatoridae and Alytidae in the form of an upper and lower bound in ACR (129 and 179 mya), and as a prior of 152 mya with normal distribution and a s.d. of 25 mya in ICR. C2 and C3: Because our combined analysis placed in both the genus Alytes and the genus Discoglossus those species occurring on the opposing sides of the Strait of Gibraltar into monophyletic groups ( D. scovazzi versus D. galganoi/jeanneae , and A. maurus versus A. dickhillenii ), we concluded that these two species pairs diverged by vicariance after the last direct land connection between Iberia and North Africa had severed, that is, after the Messinian Salinity Crisis at about 5 mya. This is in full agreement with a previous time-tree analysis of Alytes, which inferred a diversification of the A. dickhillenii/maurus/muletensis clade between 2.7 and 5.6 mya [36] . We therefore constrained the divergence between the two trans-Mediterranean pairs of sister species, each with lower bounds of 5 mya and higher bounds of 7 mya (ACR) and with a normal prior at 5 mya with 2 mya s.d. (ICR). C4: Because our first exploratory analyses reconstructed unrealistically old ages for the genus Bombina compared with previous studies [16] , we constrained the split between B. orientalis and Bombina variegata at 5–17 mya in ACR, and with a normal-distributed prior at 10 mya with a large s.d. of 10 mya in ICR [35] . Morphological methods To study Hula painted frog osteology, we used X-ray microtomography and three-dimensional (3D) visualization. Four L. nigriventer specimens, preserved in ethanol, were scanned by a microtomograph (Micro-XCT 400; Xradia, California, USA) at the Weizmann Institute of Science, Israel. One of the specimens was collected in 1955 (HUJ-R-544; National Natural History Collections at the Hebrew University of Jerusalem), and others collected during 2011 (Am2572-4; National Collections of Natural History at Tel Aviv University). Two specimens were fully scanned (HUJ-R-544 and Am2572), and head scans were performed for the other two (Am2573 and Am2574). The samples were sealed in a square poly (methyl methacrylate) box, with 2 mm width windows. At the bottom of the box, a cloth soaked in ethanol ensured a saturated atmosphere around the sample that prevented it from drying out during the scan. The microtomograph includes a sealed micro-focused source, a detector mounted on a revolving head allowing the choice of linear magnifications and a CCD (charge-coupled device) camera with 2,048 × 2,048 pixels. The micro-computed tomography scans were conducted at 40 kV, 200 μA (8 W of power) and a spatial resolution of 35 μm. The data set for an acquisition consists of nine tomograms centred on different areas of the sample, each of them including 500 projections taken over 180°, with an exposure time of 5 s per projection. Under this setup, at a linear magnification of × 0.5, scanning each individual took about 30 h. The volumes of the nine regions were reconstructed separately with specialized volume reconstruction software (Xradia, California, USA). The 3D images were generated with 16-bit precision and subsequently converted into 8 bit for visualization. Three-dimensional processing and rendering were obtained after semi-automatic segmentation of the skeleton using surface and volume rendering in AVIZO 7.01 (VSG, SAS, Merignac, France; http://www.vsg3d.com ). We studied 22 osteological characters, identifiable on non-articulated specimens of extinct and extant Alytidae taxa ( Supplementary Table S2 ). Character choice was based on Clarke’s [19] comparative morphology of extant Discoglossus , with some adjustments made based on personal observations and previous studies [18] , [20] , [37] , [38] , [39] . Character states for the osteological traits were determined by us for extant and fossil L. nigriventer , and based on literature records and museum specimens for the other fossil and recent Alytidae ( Eodiscoglossus , Callobatrachus , Wealdenbatrachus , Kizylkuma , Paradiscoglossus , Paralatonia , Latoglossus , Latonia , Discoglossus, Alytes, Bombina and Barbourula ; Supplementary Note 1 ). Because D. montalentii had some distinct characters from the other Discoglossus species, we defined it as separate taxon for phylogenetic analysis, whereas other Discoglossus species were merged because of their osteological similarity. Phylogenetic reconstruction on osteological characters used Bayesian inference [31] (MrBayes, 50 6 generations with 10 6 burn-ins) and maximum parsimony [40] (PAUP 4.0, all characters unordered, treating multiple states in one or several taxa as polymorphism and calculating 1,000 bootstrap replicates). We also used logistic regression to calculate the probability of presence of an additional set of nine osteological characters common in extant L. nigriventer , extant Discoglossus species, fossil L. nigriventer, Latonia gigantea and Latonia ragei ( Supplementary Table S3 ). The matrix of presence/absence of morphological characters, composed from skeletons of recent species and non-articulated bones of fossil species, was fitted to a fully factorial logistic model with species and character as the main effects. Accession numbers: Sequences have been deposited in NCBI GenBank Nucleotide database under accession numbers KC867706 – KC867711 . How to cite this article: Biton, R. et al . The rediscovered Hula painted frog is a living fossil. Nat. Commun. 4:1959 doi: 10.1038/ncomms2959 (2013).